An exceptionally preserved arthropod cardiovascular system from the early Cambrian The assumption that amongst internal organs of early arthropods only the digestive system withstands fossilization is challenged by the identification of brain and ganglia in early Cambrian fuxianhuiids and megacheirans from southwest China. Here we document in the 520-million-year-old Chengjiang arthropod Fuxianhuia protensa an exceptionally preserved bilaterally symmetrical organ system corresponding to the vascular system of extant arthropods. Preserved primarily as carbon, this system includes a broad dorsal vessel extending through the thorax to the brain where anastomosing branches overlap brain segments and supply the eyes and antennae. The dorsal vessel provides segmentally paired branches to lateral vessels, an arthropod ground pattern character, and extends into the anterior part of the abdomen. The addition of its vascular system to documented digestive and nervous systems resolves the internal organization of F. protensa as the most completely understood of any Cambrian arthropod, emphasizing complexity that had evolved by the early Cambrian. F uxianhuia protensa Hou, 1987, is among the most agreed upon representative of the euarthropod stem group. Its placement crownwards of anomalocaridids and bivalved arthropods such as Canadaspis refers especially to its head tagmosis and appendicular structures [1] , [2] , [3] , [4] , [5] , [6] and this phylogenetic position has been retrieved in comprehensive cladistic analyses [7] . Documentation of its brain and optic neuropils rather unexpectedly introduced similarities to crown-group euarthropods [8] , in particular to members of the Mandibulata. The exoskeletal and appendicular morphologies of F. protensa have been studied in detail, and this taxon remains the Cambrian arthropod with the most detailed information on the brain and its connections to segmental structures in the head [6] , [8] . Various specimens also reveal anatomical details of the gut [4] , [5] , [6] . An exceptional specimen of F. protensa , YKLP 11335, revealing a previously unknown internal organ system, was collected from the Yu’anshan Member of the Heilinpu Formation (Cambrian Series 2, Stage 3), in Yunnan Province, China. Like other Chengjiang deposits, this is characterized by the alternation of event and background claystone layers, representing two distinct taphonomic facies [9] , [10] . Ultra-fine-grained event claystone layers generally correspond to rapid sediment deposition that resulted in better preservation of soft-bodied fossils, while interbedded background layers are interpreted as hemipelagic deposits consisting predominantly of indeterminate algae, organic elements and a few other poorly preserved fossils [11] . The specimen central to the present account derives from such a background layer and has undergone significant decay like most fossils from these beds. Here we describe evidence for exceptional preservation of what are interpreted as cardiovascular structures in F. protensa , permitting detailed anatomical and phylogenetic comparisons between this Cambrian species and extant arthropods. Morphological description The dorsoventrally flattened specimen ( Fig. 1e ) can be clearly identified as F. protensa ( Fig. 1a–d ) by its characteristic outline, showing a semicircular head shield, a broad thorax composed of 14 post-cephalic tergites falling within the known range of 13–15 post-cephalic tergites for F. protensa [2] , [6] , and an abruptly narrowed abdomen. The posterior end of the specimen is incomplete and missing the last four segments of the abdomen and the telson. Three additional small thoracic tergites situated beneath the head shield of F. protensa [2] , [6] are not seen in this specimen due to dorsal-side-up preservation. While most detailed structures were not observed, a complex, bilaterally symmetrical structure was preserved as a distinct black to dark grey colouration within the beige-coloured, partly decayed exoskeleton ( Figs 1e and 2a ). Element mapping by energy-dispersive X-ray spectroscopy revealed this organ system to be preserved as a carbon film ( Fig. 2b ). Some areas of the carbon film, particularly in the abdomen and to a lesser degree in the head, are correlated with an additional weak iron signal ( Fig. 2c ). This structure is identified as an internal organ system, as it does not correspond to any known external features of F. protensa , which are poorly preserved in this specimen. The precise bilateral symmetry, the extension from head to abdomen and the association with other segmental structures (see below) all indicate that this structure is not a taphonomic artefact. 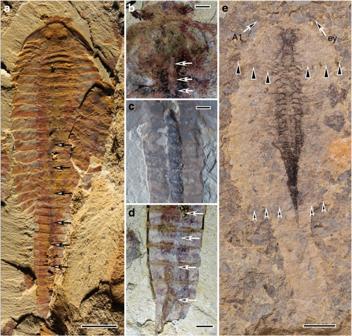Figure 1: Gut–cardiovascular comparisons ofFuxianhuia protensa. (a) Dorsal view ofF. protensa(YKLP 11336) showing disposition of gut (arrows); (b) anterior delimitation of gut at mouth opening (arrows; YKLP 11337); (c) filled gut within abdominal segments Ab1–7 (YKLP 11338); (d) empty gut (arrowed; YKLP 11339), abdominal segments Ab9–14; and (e) overview of cardiovascular system (YKLP 11335). Left antenna (A1) and right eye (ey) resolvable, as are posterior margin of head shield (top arrowheads) and posterior limit of the thorax (bottom arrowheads). Scale bar, 5 mm (a); 1 mm (b–d); 4 mm (e). Figure 1: Gut–cardiovascular comparisons of Fuxianhuia protensa . ( a ) Dorsal view of F. protensa (YKLP 11336) showing disposition of gut (arrows); ( b ) anterior delimitation of gut at mouth opening (arrows; YKLP 11337); ( c ) filled gut within abdominal segments Ab1–7 (YKLP 11338); ( d ) empty gut (arrowed; YKLP 11339), abdominal segments Ab9–14; and ( e ) overview of cardiovascular system (YKLP 11335). Left antenna (A1) and right eye (ey) resolvable, as are posterior margin of head shield (top arrowheads) and posterior limit of the thorax (bottom arrowheads). Scale bar, 5 mm ( a ); 1 mm ( b – d ); 4 mm ( e ). 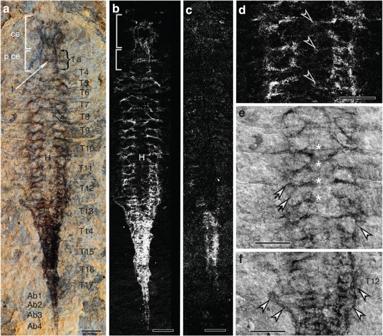Figure 2: Cardiovascular system (CVS) ofF. protensa. (a) Image of whole cardiovascular system showing broad heart (H) extending between thoracic tergites T7–T14. The CVS tapers from the level of T13 to become reduced to a single vessel at abdominal tergite Ab3 that fades to invisibility at level of Ab4. Cerebral (ce) and post-cerebral (p ce) CVS stem from paired frontal arteries (f a, bracketed upper right) that are connected by a stout heterolateral vessel (arrowed 1); (b) energy-dispersive X-ray spectroscopy (EDX) showing CVS represented by a carbon film; (c) EDX resolves Fe at the level of T13–T17; (d) enlargement of EDX between T10 and T12 demonstrating intense puncta (arrowheads) flanked by fine collateral, together interpreted as ventral projecting vessels; (e) enlargement of heart and lateral vessels between T7 and T11 demonstrating broad origins (asterisks) of lateral vessels bifurcating into main flanking arteries (at arrowheads); and (f) CVS at T11–T13 showing well preserved traces of main flanking arteries (arrowheads). Scale bar, 2 mm. Full size image Figure 2: Cardiovascular system (CVS) of F. protensa . ( a ) Image of whole cardiovascular system showing broad heart (H) extending between thoracic tergites T7–T14. The CVS tapers from the level of T13 to become reduced to a single vessel at abdominal tergite Ab3 that fades to invisibility at level of Ab4. Cerebral (ce) and post-cerebral (p ce) CVS stem from paired frontal arteries (f a, bracketed upper right) that are connected by a stout heterolateral vessel (arrowed 1); ( b ) energy-dispersive X-ray spectroscopy (EDX) showing CVS represented by a carbon film; ( c ) EDX resolves Fe at the level of T13–T17; ( d ) enlargement of EDX between T10 and T12 demonstrating intense puncta (arrowheads) flanked by fine collateral, together interpreted as ventral projecting vessels; ( e ) enlargement of heart and lateral vessels between T7 and T11 demonstrating broad origins (asterisks) of lateral vessels bifurcating into main flanking arteries (at arrowheads); and ( f ) CVS at T11–T13 showing well preserved traces of main flanking arteries (arrowheads). Scale bar, 2 mm. Full size image In overall appearance, the post-cephalic part of the organ system comprises a bilaterally symmetric arrangement of dark, segmentally paired extensions originating from a broad spindle-shaped midline structure bounded by blurred margins extending between the thoracic tergites T7 and T14 ( Fig. 2a ). This structure is punctuated at its midline by carbon deposits ( Fig. 2a,b and d ) that relate to oblique carbon film extensions ( Fig. 2d ). The entire system in the trunk gives rise to segmentally arranged lateral extensions that originate from the midline structure, which we interpret as the heart, and its anterior and posterior continuation. Where most clearly preserved, these lateral extensions originate as funnel-shaped profiles (asterisks in Fig. 2e ) that then project laterally before bifurcating into two tributaries (arrowed in Fig. 2e ). On each side of the body the tributaries merge with an antero-posterior artery, the traces of which are best preserved between thoracic tergites T11 and T14 (arrowheads in Fig. 2e,f ). The lateral extensions have a one-to-one relationship to tergites in the anterior part of the thoracic trunk (around T4–T11), but inexactly approximate two per tergite by the middle of the thorax, corresponding to the spacing of appendages in this species [2] , [6] . The structure becomes even more densely spaced from the posterior thorax to the anterior abdomen. The whole organ system tapers posteriorly from thoracic tergites T13–T17, subsequently reduced to a single midline extension from T17 as far as abdominal segment Ab4 ( Fig. 2a ). The tapering section appears much darker than other structures due to the apparent convergence of its components, although the midline regions and its pair of flanking extensions can still be recognized. Posteriorly the signal indicative of the dorsal vessel fades to pale grey and is thereafter unresolved caudally from abdominal segment Ab5. Paired frontal arteries (f a in Fig. 2a ) originate at the level of thoracic tergite T4 to extend forward beneath the cephalic shield. These provide an elaborate system of tributaries and anastomoses ( Figs 3a , 4 and 5a ). The complete organ system is interpreted as a largely intact vascular system in F. protensa . Because in the head vascular structures clearly correlate to cerebral structures ( Figs 3b,c and 5b,c ), their arrangements are best understood with reference to the brain of this species [8] . The following description thus reflects this relationship. 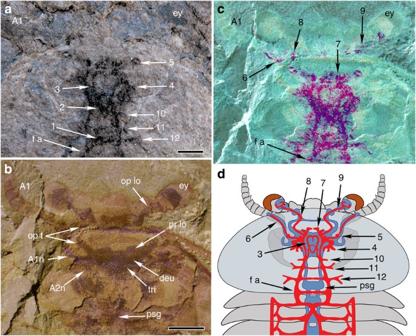Figure 3: Cerebral CVS and brain ofF. protensa. (a) Colour segmentation enhancement of the CVS in YKLP 11335. Numbers refer to descriptions in the text. Remnants of the first antenna (A1) and eye (ey) indicated; (b) brain and first post-stomodeal ganglion (YKLP 15006) showing optic lobes (op lo), optic tracts (op t), protocerebral lobes (pr lo) and the roots of the first (antennal) and second post-ocular appendage nerve (A1n, A2n). The deuto- and tritocerebrum are indicated, as is the first post-stomodeal ganglion (psg); (c) overlap of cerebral CVS (magenta, colour substitution of CVS ina) and nervous system (colour inverted fromb); (d) reconstruction of the head and anterior part of thorax (red, cardiovascular system from YKLP 11335; blue, nervous system from YKLP 15006)8. To avoid overcrowding, the three anteriormost thoracic tergites overlain by the cephalic shield are omitted. Numbers refer to vascular structures in the head relating to the location of the brain and nerve cord (arrowed 1–5, 7, 10–12), antennae and optic lobes (arrowed 6, 8, 9). Scale bar, 1 mm. Figure 3: Cerebral CVS and brain of F. protensa . ( a ) Colour segmentation enhancement of the CVS in YKLP 11335. Numbers refer to descriptions in the text. Remnants of the first antenna (A1) and eye (ey) indicated; ( b ) brain and first post-stomodeal ganglion (YKLP 15006) showing optic lobes (op lo), optic tracts (op t), protocerebral lobes (pr lo) and the roots of the first (antennal) and second post-ocular appendage nerve (A1n, A2n). The deuto- and tritocerebrum are indicated, as is the first post-stomodeal ganglion (psg); ( c ) overlap of cerebral CVS (magenta, colour substitution of CVS in a ) and nervous system (colour inverted from b ); ( d ) reconstruction of the head and anterior part of thorax (red, cardiovascular system from YKLP 11335; blue, nervous system from YKLP 15006) [8] . To avoid overcrowding, the three anteriormost thoracic tergites overlain by the cephalic shield are omitted. Numbers refer to vascular structures in the head relating to the location of the brain and nerve cord (arrowed 1–5, 7, 10–12), antennae and optic lobes (arrowed 6, 8, 9). Scale bar, 1 mm. 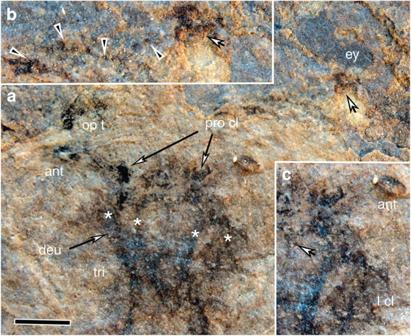Figure 4: Cerebral CVS ofF. protensa. (a) Main panel: origin of left optical artery (op a) at the protocerebral cluster (pro cl). (b) Upper inset: right optical artery trajectory (at arrowheads) to semicircular sinus at the level of the second optic neuropil beneath the eye (ey). Origin of antennal arteries (ant) demonstrate overall symmetry of the cerebral CVS, as do two parallel ascending vessels (asterisks) ascending from the tritocerebral segment (tri) through the deutocerebrum (deu). Asymmetry of the left and right lateral clusters (l cl) in the deutocerebrum results in loss of definition on the left. (c) Lower left inset: details of l cl anastomizations and the caudally extending midline vessel (arrowed) at protocerebrum. Scale bar, 1 mm. Full size image Figure 4: Cerebral CVS of F. protensa . ( a ) Main panel: origin of left optical artery (op a) at the protocerebral cluster (pro cl). ( b ) Upper inset: right optical artery trajectory (at arrowheads) to semicircular sinus at the level of the second optic neuropil beneath the eye (ey). Origin of antennal arteries (ant) demonstrate overall symmetry of the cerebral CVS, as do two parallel ascending vessels (asterisks) ascending from the tritocerebral segment (tri) through the deutocerebrum (deu). Asymmetry of the left and right lateral clusters (l cl) in the deutocerebrum results in loss of definition on the left. ( c ) Lower left inset: details of l cl anastomizations and the caudally extending midline vessel (arrowed) at protocerebrum. Scale bar, 1 mm. 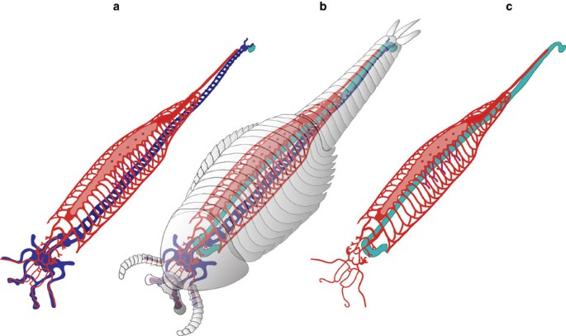Figure 5: Reconstructions ofF. protensa. (a) Cardiovascular system (red) shown in relation to the brain and central nervous system (blue); (b) whole reconstruction, with brain and segmental ganglia (blue) shown in relation to serial arrangements of tergites. The reconstruction of the vascular system assumes that posterior abdominal extensions of the dorsal vessel are likely present although these are not defined by carbon traces in the fossil. The reconstruction of the nervous system infers that paired nerves are associated with the telson. As described elsewhere1,2,6, tergites do not reflect true metamerism, there being >1 ganglion coincident with each tergite from T7. Likewise, lateral vessels occur one per tergite frontally in the thorax but are more crowded further towards the rear; (c) cardiovascular system (red) in relation to the gut (green). Full size image Figure 5: Reconstructions of F. protensa . ( a ) Cardiovascular system (red) shown in relation to the brain and central nervous system (blue); ( b ) whole reconstruction, with brain and segmental ganglia (blue) shown in relation to serial arrangements of tergites. The reconstruction of the vascular system assumes that posterior abdominal extensions of the dorsal vessel are likely present although these are not defined by carbon traces in the fossil. The reconstruction of the nervous system infers that paired nerves are associated with the telson. As described elsewhere [1] , [2] , [6] , tergites do not reflect true metamerism, there being >1 ganglion coincident with each tergite from T7. Likewise, lateral vessels occur one per tergite frontally in the thorax but are more crowded further towards the rear; ( c ) cardiovascular system (red) in relation to the gut (green). Full size image The frontal arteries are connected by a broad transverse channel (arrowed 1, Figs 2a and 3a ) in the post-cerebral area of the head (p ce, Fig. 2a ), providing paired lateral branches (arrowed 12, Fig. 3a,d ) at the level of the fourth cephalic segment, corresponding to the assumed location of the first post-stomodeal ganglion (psg, Fig. 3b ). Forward of this, in the cerebral area (ce, Fig. 2a ) at the approximate level of the brain’s tritocerebrum, the frontal vessels are connected by a V-shaped anastomosis (arrowed 2 in Fig. 3a ). The upper arms of the V project forwards and then recurve downwards to fuse at the midline, thereby providing an obcordate profile (arrowed 3 in Fig. 3a,d ). At their point of closure the arms provide a single short artery extending posteriorly along the midline of the brain ( Fig. 3a,c and d , arrow, lower right inset; Fig. 4 ). The paired frontal arteries provide a crozier-shaped extension with short branches each side of the brain (lateral cluster; arrowed 4 in Fig. 3a,d ) that broadens to flank the lateral deutocerebrum (deu, Fig. 3b ). The shapes of the left and right clusters have not been preserved symmetrically, however, because the left frontal artery extends slightly further forward than the right to provide a diffuse, palmate trace (leftmost asterisk, Fig. 4 ). We interpret both extensions as equivalent, their asymmetry a result of taphonomic distortion. In other respects, structures and traces of vessels further forward, at the level of the protocerebral lobes, show a high degree of symmetry, including the origin of the paired antennal arteries (arrowed 5 in Fig. 3a,d ; ant, Fig. 4 ), one of which extends into the first annulus of the left antenna (arrowed 6, Fig. 3c,d ). Traces of optical arteries are also visible originating from two dense areas, here termed the protocerebral clusters (arrowed 7, Fig. 3c,d ; pro cl, Fig. 4 ). The left optical artery (arrowed 8, Fig. 3c,d ) is seen to follow the course taken by the brain’s optic tract (op t, Figs 3b and 4 ). The right optical artery (arrowed 9, Fig. 3c,d ) is resolved extending out to the eye (ey, Fig. 3a–c ), here also preserved as a distinct trace. The optical artery (arrowheads, Fig. 4 ) forms a curved terminus at the level of the optic lobe ( Fig. 3d , arrow at ey, Fig. 4 ). Other smaller lateral arteries extend from the frontal arteries behind the brain proper at the level of the mouth opening (arrowed 10, 11, Fig. 3a,d ). Identity of the organ system The present organ system is distinct from the digestive and nervous system. Digestive tracts show morphological diversity in different Cambrian arthropods, many evidencing systems of diverticula in the head and trunk [12] , [13] . In contrast, previous studies [5] , [6] and the present observations demonstrate that F. protensa has a simple tubular gut extending from the mouth to the last segment of the abdomen ( Figs 1a–d and 5a ). Unlike, for example, leanchoiliids [12] or naraoiids [13] , there are no gut diverticula in F. protensa . Elongate pellet-like fill has been found in most preserved guts of F. protensa , providing a three-dimensional relief and colouration that distinguishes the alimentary canal from its surrounding tissue. However, even an empty gut can be well resolved as far as the terminal anus ( Fig. 1d ). Several specimens show that the gut has a slightly more tortuous trajectory within the anterior thorax ( Fig. 1a ). The central nervous system of F. protensa is also distinct from the present organ system ( Fig. 4c ). As described previously [8] , the cerebral ganglia are preserved as a contiguous bilaterally symmetric structure comprising three segments, each defined by its paired nerve tracts associated with the protocerebral optic lobes and the deutocerebral antennae (A1) and short tracts [8] , terminating above the location of the roots of the paired scimitar-like second post-ocular appendages (A2) ( Fig. 3c ) disposed ventrally beneath the head [1] , [14] . Ventral nerve cords in the related fuxianhuiid Chengjiangocaris kunmingensis are preserved as paired connectives linking segmentally discrete ganglia [14] . There is no basis for ambiguity between the structures in YKLP 11335 and the stomatogastric nervous system, such as that described from the cephalocarid Hutchinsoniella macracantha [15] . The stomatogastric nervous system comprises slender median and lateral neurite bundles with collaterals extending through most of the trunk. However, no branches extend anteriorly beyond the mouth opening nor are they associated with other head structures [15] . Were a delicate stomatogastric nervous system preserved in YKLP 11335, it would be expected that robust components of the central nervous system would likewise be preserved, but no trace of these is seen. Comparisons with extant arthropods identify the present organ system as a cardiovascular system ( Fig. 5a–c ). Although preserved flattened, its broad midline structure corresponds to a medial heart from which extend systems of anterior, lateral and posterior arteries, comparable to those observed in many aquatic and terrestrial arthropods. Although adopting diverse shapes in extant arthropods [16] , the heart provides discrete arrangements of segmentally distributed vessels that supply other organ systems, such as the brain and appendages. The same principle arrangement of the cardiovascular system is recognized across extant Arthropoda. Comparison with fossil and extant vascular systems There are relatively few prior studies on circulatory systems in fossil arthropods. The finely branched genal caecae in various trilobites, including some Cambrian species, have been suggested to have a respiratory and/or circulatory function [17] , [18] , [19] . Assumed integumental haemolymph networks were described in the carapace valves of Cambrian bradoriids and a bivalved arthropod from the Burgess Shale [20] and compared with circulatory systems of recent ostracods [21] . However, these previous studies did not refer to the vascular system within the body. An exception is the Burgess Shale arthropod Marrella splendens , in which reflective areas have been interpreted as cardiovascular, suggesting a heart localized in the cephalon and arteries extending into cephalic spines and the appendages [22] . However, this putative system is difficult to compare with extant arthropods, partly due to its peculiar morphology and controversy over the affinities of Marrella to either Chelicerata [2] or Mandibulata [7] . In contrast, cardiovascular traces preserved in the present specimen of F. protensa demonstrate a number of correspondences with vascular arrangements in extant mandibulates. In scutigeromorph centipedes, for example, the anterior aorta gives off a trunk that splits into two ventrally extending, shorter, sac-like contractile ‘aortic diverticles’ [23] , the placement of which corresponds to expansions from the lateral arteries at the level of the deutocerebrum in F. protensa (arrowed 4, Fig. 3a,d ). As occurs in branchiopod and stomatopod crustaceans [24] , the heart in F. protensa provides paired lateral vessels in successive thoracic segments. It is these branches that merge with the long antero-posterior flanking arteries ( Figs 2f and 5a ). In most crustaceans, a single anterior artery extends forward from the heart [25] , whereas in F. protensa the equivalent anterior extension is extremely short and broad thereafter providing an aortic arch, beneath the first thoracic tergite T1, from which extend the paired frontal arteries into the cephalic region ( Fig. 5a,b ). The frontal arteries ( Figs 2a and 3a ) provide anastomizations and vessels, the arrangements of which most closely resemble those relating to the cerebral ganglia of malacostracans [26] , [27] . Notable in both F. protensa and Malacostraca are antennal and optic arteries supplying the first antennae and eye stalks; in F. protensa the optic arteries have forked terminations at optic neuropils ( Figs 3a,c and 4 ), such as those of decapods. Optical arteries and elaborate cephalic arteries are likewise prominent in other malacostracans [27] . Because the fossilized cardiovascular system in F. protensa is preserved flattened, determining whether there is a ventral vessel is challenging. However, the presence of segmentally arranged puncta at the midline of the dorsal vessel ( Fig. 2d ), from which extend barely discernable lateral branches, suggests a system of downward-projecting midline vessels analogous to those observed in mysid crustaceans (Malacostraca) [26] . The similarity of the cardiovascular system of F. protensa with those of mandibulates contrasts with comparisons with xiphosurans, which resolve few correspondences other than a prominent dorsal heart, which gives off short pairs of lateral cardiac arteries (four in the case of Limulus polyphemus ) that merge with vessels flanking the pericardium [28] . In L. polyphemus , arches of the anterior aorta extend to within the brain’s massive corpora pedunculata [29] , and an anterior artery expands into a complex system of ventral midline and bilateral arteries [28] . These are associated with the gut, appendages and ventral nerve cord. Pairs of segmentally arranged lateral arteries supply the chelicera, limbs and book lungs [28] . These arrangements have no obvious correspondence to arteries in F. protensa or in described extant mandibulates [16] , [25] , [27] . If the segmental organization of lateral vessels observed in F. protensa ( Fig. 5b ) represents a ground pattern of euarthropod cardiovascular systems, consistent with the placement of Fuxianhuiida as sister group to Megacheira (an extinct group of great-appendage arthropods) plus crown-group Euarthropoda [7] , then clearly there is evidence for many variations of divergence, as well as secondary reductions, of cardiovascular elements in extant mandibulates. Most obvious is the absence in chilopods [30] , symphylans and in most malacostracans of iterated lateral vessels from the dorsal vessel. However, iterated lateral arteries from the dorsal vessel are known in diplopods [31] and in some malacostracans and branchiopods [24] , [25] , and their presence in xiphosurans, pulmonate arachnids and insects [16] , [25] argues that their presence in F. protensa is a ground pattern character for euarthropods as a whole. The observation that F. protensa shares with Tetraconata a tripartite supraesophageal brain [8] indicates either an early evolution of the crustacean cerebral ground pattern or convergent evolution of an organization typifying extant crustaceans. The vascular system of F. protensa described here represents the earliest complete cardiovascular system known from any fossil arthropod. The identification of a cardiovascular system that compares best with those of extant mandibulates adds novel characters for phylogenetic analysis. These, and earlier results [8] , are consistent with a more crownwards position of fuxianhuiids than had been inferred from external characters of tagmosis and appendage structure. The cephalic parts of the vascular system of F. protensa are strikingly similar to those of Lophogastrida [26] and Euphausiacea [32] , which belong, respectively, to the malacostracan superorders Peracarida and Eucarida. As both these two extant groups are deeply nested in the Mandibulata, the similarity of vascular systems between them and F. protensa is likely to be the result of functional convergence. Such a rich system of arteries in F. protensa associated with its brain suggests a demand for oxygen required by networks integrating information from well-developed visual and antennal sensory systems, thereby substantiating the view that this taxon was a highly mobile forager employing active vision and olfactory perception. These findings add to an emerging picture that arthropods had evolved sophisticated sensory adaptations and neural networks supplied by elaborate cardiovascular systems by the main burst of the Cambrian explosion [33] . Material All investigated specimens of F. protensa (YKLP 11335–11339) are housed at the Yunnan Key Laboratory for Palaeobiology, Yunnan University, Kunming, China. Locality and horizon All specimens were collected from the Yu’anshan Member of the Heilinpu Formation (Cambrian Series 2, Stage 3) at Ercaicun village, Haikou, Yunnan Province, China. Imaging Digital images of the specimen were captured with a Leica DFC5000 camera attached to a Leica M205C photomicroscope and were processed in Adobe Photoshop CS5. Elemental analyses were obtained using energy-dispersive X-ray microscopy with a LEO 1455VP scanning electron microscope, at 12 kV accelerating voltage and 12 Pa chamber pressure. The final carbon and iron maps were montaged from individual maps with Adobe Photoshop CS5. Reconstructions Reconstructions of organ systems made using Adobe Illustrator are based on specimens preserving the gut (YKLP 11336, YKLP 11337, YKLP 11338 and YKLP 11339), the brain (YKLP 15006 (ref. 8 )), segmental nervous system [14] and vascular system (YKLP 11335) with references to described external morphology [1] , [2] , [3] , [4] , [5] , [6] . How to cite this article: Ma, X. et al . An exceptionally preserved arthropod cardiovascular system from the early Cambrian. Nat. Commun. 5:3560 doi: 10.1038/ncomms4560 (2014).